Active and stable carbon nanotube/nanoparticle composite electrocatalyst for oxygen reduction Nanostructured carbon-based materials, such as nitrogen-doped carbon nanotube arrays, Co 3 O 4 /nitrogen-doped graphene hybrids and carbon nanotube–graphene complexes have shown respectable oxygen reduction reaction activity in alkaline media. Although certainly promising, the performance of these materials does not yet warrant implementation in the energy conversion/storage devices utilizing basic electrolytes, for example, alkaline fuel cells, metal-air batteries and certain electrolysers. Here we demonstrate a new type of nitrogen-doped carbon nanotube/nanoparticle composite oxygen reduction reaction electrocatalyst obtained from iron acetate as an iron precursor and from cyanamide as a nitrogen and carbon nanotube precursor in a simple, scalable and single-step method. The composite has the highest oxygen reduction reaction activity in alkaline media of any non-precious metal catalysts. When used at a sufficiently high loading, this catalyst also outperforms the most active platinum-based catalysts. Electrochemical reduction of oxygen in basic media is an important reaction for electrochemical devices directly related to efficient energy conversion and storage: fuel cells (operating with either liquid or polymer electrolytes), metal-air batteries and certain electrolysers (for example, chlor-alkali ones). Among those devices, a lithium (Li)-air secondary battery, potentially the most promising metal-air battery known, with a storage capacity approximately ten times that of the state-of-the-art Li-ion battery, can find application in hybrid electric vehicles and energy storage for intermittent sources of electricity, such as solar and wind [1] . In turn, the replacement of hydrogen-evolving cathode with an air cathode in chlor-alkali electrolysers is expected to reduce the energy consumption in the United States by close to 1% (thanks to lowering of the cathode-operating overpotential by more than 1.2 V ( E° values of −0.828 V and 0.401 V, respectively)) [2] . A successful large-scale implementation of these technologies depends, however, on the advent of active, stable and selective oxygen reduction reaction (ORR) catalysts, preferably free of precious metals. To date, platinum (Pt) has shown the highest ORR activity in alkaline media. As a potential Pt replacement, silver (Ag) has been more thoroughly studied in comparison with other catalysts because of its relatively high activity, abundance and low cost. However, the ORR half-wave potential ( E 1/2 ) in rotating-disk electrode (RDE) polarization studies is by ca. 0.2 V lower for Ag than for Pt [3] , [4] . Carbon-based catalysts with promising ORR activity in alkaline electrolytes have also been demonstrated [5] , [6] . Although details of the ORR mechanism on such catalysts are yet to be fully understood, the adsorption of oxygen and formation of superoxide through a one-electron reduction (O 2 +e − ←[O 2(ads) ] − ) have generally been viewed as initial ORR steps [5] , [6] , with O 2 adsorption proposed by Morcos and Yeager [5] to be the rate-determining step. Thanks to preferred O 2 adsorption on the exposed edge of graphene rather than the basal plane itself, the edges show high ORR activity comparable to that of Pt, while basal planes remain virtually ORR inactive [5] , [6] . N-doping into carbon nanotubes (CNTs) has been found to increase ORR activity in alkaline media by ca. 0.2 V at the E 1/2 (refs. 7 , 8 ). Doped nitrogen species increase the graphene edge presence by facilitating the formation of pentagonal defects in hexagonally arranged carbon atoms, causing disruption to the graphene structure, and by introducing irregularities to the curvature in the graphene stacking [9] , which eventually lead to enhanced ORR activity [7] . As these original findings were published [7] , [8] , various N-doped carbon catalysts, including CNTs [10] , [11] , [12] , graphene [13] , [14] , mesoporous carbon [15] , [16] and particulate [17] , have been studied as a possible replacement for Pt. However, only vertically aligned N-containing CNTs (VA-NCNTs) have so far shown E 1/2 values comparable to those measured with Pt/C catalysts [8] . VA-NCNTs are typically grown on a quartz substrate by chemical vapour deposition. A free-standing VA-NCNT film is obtained following a treatment with hydrofluoric acid that allows the catalyst film to be peeled off the substrate [8] . This expensive and tedious synthesis path precludes large-scale fabrication of the catalyst, rendering VA-NCNTs non-competitive with Pt-based catalysts. Here we introduce a new type of N-doped nanostructured carbon-based catalyst, synthesized using iron acetate, Fe(CH 3 -COO) 2 , as an iron precursor and cyanamide, NCNH 2 , as a nitrogen precursor for iron-activated, N-doped catalyst, in which carbon phase is made up of a CNT/carbon nanoparticle (CNP) composite. This catalyst, labelled N-Fe-CNT/CNP, can be synthesized via a simple and scalable method using Fe, not only to induce ORR activity but also to catalyse the CNT growth. This composite catalyst shows the highest ORR activity in alkaline media of any nanostructured carbon-based catalysts [8] , [10] , [13] . When used at a sufficiently high loading, this catalyst also outperforms the most active Pt-based catalysts [18] , [19] , [20] , [21] . Synthesis A solution of 3.5 g of cyanamide and 1.0 g of iron acetate in ethanol was first stirred for 3 h at 60 °C. One gram of oxidized carbon powder (Black Pearls 2000 pretreated in 70% nitric acid at 80 °C for 8 h) was then added to the solution and stirred at 60 °C overnight. Finally, the solvent was evaporated at 45 °C and remaining powder converted into the N-Fe-CNT/CNP composite catalyst by a heat treatment at 950 °C in nitrogen for 1 h. To remove a redundant phase, mainly unreacted metallic iron and iron compounds, the N-Fe-CNT/CNP composite catalyst was preleached in 0.5 M H 2 SO 4 at 80 °C for 8 h. In the final step, the catalyst was heat-treated for a second time under the same conditions as during the first heat treatment. Although cyanamide has been primarily used as a source of graphitic-C 3 N 4 (ref. 22 ), one of the important accomplishments of this work is the discovery that cyanamide can also serve as a CNT precursor. Characterization High-resolution transmission electron microscopy image of as-obtained N-Fe-CNT/CNP catalyst shows CNTs, ca. 20–30 nm in outer diameter and ca. 10 μm in length, homogeneously distributed in the CNP phase ( Fig. 1a and Supplementary Fig. S1 ). The image of a CNT tip in Fig. 1b reveals iron encapsulated in several graphene nanoshells, the result of Fe-catalysed growth of CNTs. Iron particles are encapsulated in graphene nanoshells either at the tip or inside CNTs ( Supplementary Fig. S2a–d ). In some instances, iron can be encapsulated in the graphene nanoshells that are not part of the nanotubes ( Supplementary Fig. S2e ), which suggests that the encapsulation of iron into graphene nanoshells can be the first step of the CNT growth. Bamboo-like ‘joints’ ( Fig. 1c and Supplementary Fig. S2f ), also observed by others [7] , [8] , represent a typical morphological feature of N-doped CNTs synthesized in this work. The nitrogen content in the N-Fe-CNT/CNP composite catalyst, as measured by X-ray photoelectron spectroscopy (XPS), is 3.1 at% ( Supplementary Table S1 ). XPS N 1s spectra can be deconvoluted into three peaks assignable to the pyridinic (398.3 eV), pyrrolic (400.0 eV) and graphitic (401.1 eV) nitrogen atoms ( Supplementary Fig. S3 ). Although N-doping alone has been known to produce defects in the graphene stacking in CNTs [7] , [9] , the defects in the N-Fe-CNT/CNP catalyst can also be caused by CNPs obstructing linear CNT growth. The defects in graphene stacking in CNTs, resulting in the formation of O 2 adsorption sites, are believed to be an important contributing factor to high activity of carbon-based catalysts [5] , [6] , [7] . The goal of generating high number of exposed graphene edges and, consequently, a high number of active ORR sites was achieved in this work via a single-step synthesis of N-doped CNT/CNP composite catalyst. 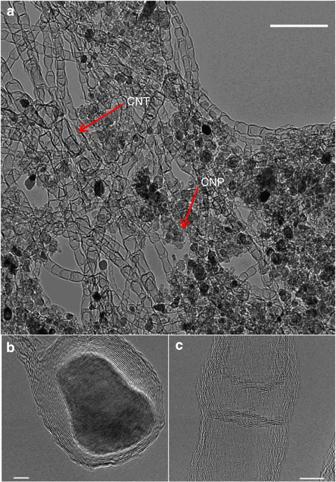Figure 1: Micrographs of carbon nanotube/nanoparticle composite. (a) High-resolution transmission electron microscopy of the N-Fe-CN/CNP composite catalyst. Scale bar, 200 nm. (b) Iron encapsulated in graphene nanoshells, Scale bar, 5 nm. (c) Typical bamboo-like defect in graphene stacking. Scale bar, 10 nm. Figure 1: Micrographs of carbon nanotube/nanoparticle composite. ( a ) High-resolution transmission electron microscopy of the N-Fe-CN/CNP composite catalyst. Scale bar, 200 nm. ( b ) Iron encapsulated in graphene nanoshells, Scale bar, 5 nm. ( c ) Typical bamboo-like defect in graphene stacking. Scale bar, 10 nm. Full size image CNT-based composites have found numerous applications, for example, in Li-ion batteries and supercapacitors [23] , [24] , all requiring high nanotube dispersion—a big technical challenge because of CNTs’ tendency to self-agglomerate. Surface functionalization via a chemical treatment is therefore often needed, which results in additional processing steps and high cost. Contrary to the commonly used approaches, the synthesis of the N-Fe-CNT/CNP catalyst allows to achieve the desired CNT dispersion in a single step, without any additional treatments. Electrochemical performance ORR polarization data recorded with the N-Fe-CNT/CNP composite catalyst in 0.1 M NaOH at an RDE are shown in Fig. 2 . The E 1/2 value measured with the catalyst at a loading of 0.2 mg cm −2 is 0.87±0.01 V ( Fig. 2a and Supplementary Fig. S4 ). For reference, the E 1/2 value for a Pt/C catalyst (20 wt% Pt/C E-TEK) at a high precious metal loading of 60 μg Pt cm −2 is 0.91 V ( Fig. 2a ), similar to the E 1/2 value measured with a single crystal of Pt (111) ( ca. 0.90 V) (ref. 3 ). Although the E 1/2 value of 0.87 V is lower than that recorded with the Pt/C reference catalyst, the onset ORR potential measured with the N-Fe-CNT/CNP composite catalyst is by ca. 40 mV higher than for Pt/C ( Fig. 2a , inset). On the basis of the onset potential values, the intrinsic ORR activity of the N-Fe-CNT/CNP composite appears to be higher than that of the Pt/C catalyst, with N-Fe-CNT/CNP suffering at higher overpotentials from a lower density of active ORR sites, reflected by a lower E 1/2 value. In agreement with these observations, an increase in the N-Fe-CNT/CNP catalyst loading at the disk from 0.2 to 1.0 mg cm −2 yields a much-improved E 1/2 value of 0.93 V, which exceeds the value measured with the Pt/C reference by ca . 20 mV ( Fig. 2a ). 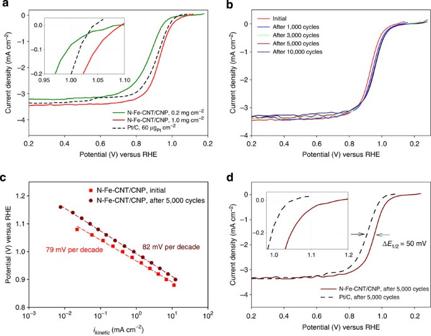Figure 2: The ORR performance of N-Fe-CNT/CNP composite and Pt/C catalysts. Steady-state RDE polarization plots obtained using 20 mV potential step and 25 s potential hold time at every step; electrolyte 0.1 M NaOH; temperature 25 °C; rotation rate 900 r.p.m. ORR at the N-Fe-CNT/CNP catalyst measured in a negative-going scan; ORR at the Pt/C catalyst measured in a positive-going scan; insets zooming on low overpotential region. (a) ORR polarization plots before cycling durability test. (b) ORR polarization plots measured during cycling durability in O2-saturated 0.1 M NaOH (cycling in the potential range 0.6–1.0 V at 50 mV s−1; N-Fe-CNT/CNP loading 1.0 mg cm−2). (c) Tafel plots for the N-Fe-CNT/CNP catalyst before and after 5,000 cycles in an O2-saturated electrolyte (Tafel slope calculated by linear regression method in the intermediate range of current densities, 10−2–101mA cm−2). (d) ORR polarization plots after 5,000 cycles in O2-saturated electrolyte. Figure 2: The ORR performance of N-Fe-CNT/CNP composite and Pt/C catalysts. Steady-state RDE polarization plots obtained using 20 mV potential step and 25 s potential hold time at every step; electrolyte 0.1 M NaOH; temperature 25 °C; rotation rate 900 r.p.m. ORR at the N-Fe-CNT/CNP catalyst measured in a negative-going scan; ORR at the Pt/C catalyst measured in a positive-going scan; insets zooming on low overpotential region. ( a ) ORR polarization plots before cycling durability test. ( b ) ORR polarization plots measured during cycling durability in O 2 -saturated 0.1 M NaOH (cycling in the potential range 0.6–1.0 V at 50 mV s −1 ; N-Fe-CNT/CNP loading 1.0 mg cm −2 ). ( c ) Tafel plots for the N-Fe-CNT/CNP catalyst before and after 5,000 cycles in an O 2 -saturated electrolyte (Tafel slope calculated by linear regression method in the intermediate range of current densities, 10 −2 –10 1 mA cm −2 ). ( d ) ORR polarization plots after 5,000 cycles in O 2 -saturated electrolyte. Full size image The ORR Tafel slope measured with the N-Fe-CNT/CNP composite catalyst is ca. 80 mV per decade ( Supplementary Fig. S5a ). This value is similar to the one determined in this work for the Pt/C catalyst in the range of intermediate current densities, 0.2–5.0 mA cm −2 ( Supplementary Fig. S5b ). A cycling durability test in O 2 -saturated solution in the potential range of 0.6–1.0 V at a scan rate of 50 mV s −1 not only shows no performance loss after 5,000 cycles but a positive shift in the E 1/2 value ( Fig. 2b ). Although advanced surface characterization techniques may be needed to elucidate the mechanism of such an activity enhancement, a similar potential shift with cycling was already observed before with non-precious metal ORR catalysts at high current densities in proton conducting fuel cells [25] . In this work, the catalyst performance stabilizes after the first 5,000 cycles, with no further ORR activity change observed during the last 5,000 cycles ( Fig. 2b ). No changes upon cycling can be seen in the voltammograms recorded in the absence of oxygen, indicating that surface properties of the catalyst are maintained during cycling ( Supplementary Fig. S6 ). During an analogous cycling test of the Pt/C reference catalyst the E 1/2 value decreases by ca. 0.01 V down to 0.90 V ( Supplementary Fig. S7 ). Chronoamperometric (constant potential) testing confirms very good stability of the N-Fe-CNT/CNP catalyst, including that at the highest current densities accessible in RDE experiments ( Supplementary Fig. S8 ). On the basis of the data recorded at 0.4 V, the stability of a N-Fe-CNT/CNP performance is better than that of a reference Pt/C catalyst. It is possible that high selectivity for the four-electron reduction of O 2 (see below) is an important contributing factor to high stability of the N-Fe-CNT/CNP catalyst. The Tafel slope of ca. 80 mV per decade, initially measured with the N-Fe-CNT/CNP, remains virtually unchanged during cycling ( Fig. 2c ). Because of a gradual increase in the non-precious metal catalyst activity and a slight decrease in the activity of the Pt/C catalyst, the initial performance gap between the two catalysts increases to ca. 50 mV at E 1/2 during cycling ( Fig. 2d ). The onset ORR potential measured with the N-Fe-CNT/CNP catalyst after 5,000 cycles increased to 1.16 V ( Fig. 2d , inset). The highest E 1/2 and ORR onset potential to date were obtained in acid electrolytes with single-crystalline Pt 3 Ni catalyst ( E 1/2 ca. 0.92 V, ORR onset potential ca. 1.0 V) [18] and nanoporous PtNi catalyst ( E 1/2 ca. 0.96 V, ORR onset potential ca. 1.05 V) [20] . Thus, the performance of the N-Fe-CNT/CNP composite catalyst developed in this work not only significantly exceeds that of any Pt-based catalyst in alkaline media but also at least matches performance of the most active Pt-alloy catalysts in acidic media (comparison made in reversible hydrogen electrode (RHE) potential scale). The volumetric activity of the N-Fe-CNT/CNP catalyst after 5,000 cycles, calculated from i kinetic in Fig. 2c , is 4.8±0.8 A cm −3 at 0.9 V. The latter value is ca. 37% higher than that obtained by Piana et al . [26] (3.5±1.0 A cm −3 ) and 50% higher than the value measured by Meng et al . [17] (3.2 A cm −3 ), but are still within the standard errors involved in the volumetric activity determination in these studies and the referenced research herein. Therefore, one should be careful making a performance superiority claim for the N-Fe-CNT/CNP catalyst based solely on the volumetric activity at 0.9 V. The true advantage of this catalyst is revealed, however, at even higher electrode potentials. Although other non-precious metal catalysts exhibit no detectable ORR activity at 1.0 V, a respectable volumetric activity of 0.32 A cm −3 is measured with N-Fe-CNT/CNP at that potential. Together with the very high onset potential value of 1.16 V, volumetric activity at 1.0 V attests to the unique performance of the N-Fe-CNT/CNP catalyst. When implemented in an alkaline fuel cell, the N-Fe-CNT/CNP catalyst is likely to allow cathode operation very close to 1.0 V. The rotating ring-disk electrode (RRDE) results are shown in Supplementary Fig. S9 where the selectivity of N-Fe-CNT/CNP for four-electron reduction of oxygen is given in terms of hydrogen peroxide yield (% H 2 O 2 ). The peroxide yield can be directly correlated with the average number of electrons transferred per O 2 molecule, n e ( n e =4−(% H 2 O 2 )/50%). In the potential range where hydrogen generation can be at all detected ( E <0.80 V), the average number of electrons transferred decreases from 4.00 (no peroxide generation) to 3.92 at the lower polarization limit of 0.20 V (and for the low catalyst loading of 0.2 mg cm −2 ), still respectable by either non-precious metal or precious metal ORR electrocatalysis standards. Unlike other carbon-based oxygen reduction catalysts, for which the onset potentials for ORR and H 2 O 2 generation coincide [8] , H 2 O 2 generation at the N-Fe-CNT/CNP catalyst in this work starts at 0.79 V, ca. 0.29 V below the ORR onset potential, a behaviour similar to that observed with Pt catalysts [3] . We developed a new N-Fe-CNT/CNP composite electrocatalyst for ORR using a synthesis method that is expected to be readily scalable to larger volumes and applicable to the synthesis of other CNT-based composites. The catalyst exhibits higher ORR activity and better stability in the alkaline electrolyte than the state-of-the-art Pt/C catalysts. Its activity also exceeds that of other non-precious metal catalysts, including the recently published VA-NCNT catalyst [8] . The N-Fe-CNT/CNP catalyst promises to replace Pt-based catalysts in alkaline media and to have an important role in enhancing the performance of alkaline fuel cells, and possibly metal-air batteries and chlor-alkali electrolysers. Electrochemical measurements RDE and RRDE measurements were performed using a CHI Electrochemical Station (Model 750b) in a standard three-electrode cell. A 5.0-mm diameter glassy carbon disk (disk geometric area 0.196 cm 2 ) and a 5.61-mm diameter glassy carbon disk with Pt ring (geometric area 0.247 cm 2 ) were used in RDE and RRDE experiments, respectively. To avoid any potential contamination of the catalyst by Pt, all experiments involving N-Fe-CNT/CNP catalysts were carried out with a graphite rod as a counter electrode in a compartment separated from the main chamber by a glass frit. A reference electrode, also separated by a glass frit, was an Ag/AgCl electrode in 3.0 M NaCl. All potentials initially measured versus the Ag/AgCl electrode were converted to a RHE scale by adding 0.966 V (the potential of the Ag/AgCl reference measured against RHE). The catalyst ink was prepared by ultrasonically blending for 1 h 10 mg of the catalyst and 40 μl of 5 wt% Nafion suspension in alcohol (Solution Technology, Inc.), in 2.5 ml solution containing isopropanol and deionized water, 4:1 by volume. Before RDE experiments, 10 μl of the solution was applied to the 0.196-cm 2 disk, resulting in a catalyst loading of 0.2 mg cm −2 . The reference Pt/C catalyst ink was prepared by ultrasonically blending for 5 min 1 mg of 20 wt% Pt/C (E-TEK) in 1 ml of deionized water. The reference catalyst loading was 60 μg Pt cm −2 . After drying the ink, 5 wt% Nafion suspension in alcohol was diluted with deionized water to attain 1:19 alcohol-to-water ratio by volume; 15 μl of that solution was then added on top of the Pt/C catalyst layer. The counter electrode in experiments involving the Pt/C reference catalyst was a platinized Pt wire. All RDE and RRDE testing was performed at a room temperature, 25±1 °C, in oxygen-saturated 0.1 M NaOH at a rotation rate of 900 r.p.m. The electrodes were activated by cyclic voltammetry in oxygen-saturated electrolyte at a scan rate of 50 mV s −1 and potential range of 0.0–1.2 V versus RHE. ORR polarization plots with non-precious metal catalyst were recorded under steady-state conditions, starting at the open cell potential (1.1–1.3 V, depending on the catalyst loading used) down to 0.0 V versus RHE, using a 0.02 V step and a potential hold time of 25 s. A 120-s potential hold at the open cell potential preceded every ORR polarization experiment. Because of the irreversible nature of the Pt surface hydroxide/oxide formation, polarization plots with the Pt/C catalyst were recorded using a positive-going scan, from 0.0 to 1.1 V versus RHE, under, otherwise, the same conditions as those used in testing of N-Fe-CNT/CNP composite catalysts. The ring collection efficiency in RRDE experiments was 0.36, as measured using a Fe(CN) 6 4−/3− redox couple. The ring potential was set to 1.3 V versus RHE. Volumetric activity was calculated from the product of mass activity (A g −1 ) and effective catalyst density (g cm −3 ). The mass-transport-corrected kinetic current density was obtained from Tafel plots. A relatively conservative value of the effective catalyst density of 0.4 g cm −3 was used to convert mass activity into volumetric activity. The catalyst effective density was determined based on X-ray tomography and scanning electron microscopy images. Virtually identical effective density values were published by Gasteiger et al . [27] and Lefèvre et al . [28] Physical characterization XPS measurements were performed on a Kratos Axis Ultra spectrometer using monochromatic Al Kα line (1,486.6 eV) as an X-ray source. High-resolution transmission electron microscopy images were taken on a JEOL 2010 microscope operating at 200 kV. How to cite this article: Chung, H. T. et al . Active and stable carbon nanotube/nanoparticle composite electrocatalyst for oxygen reduction. Nat. Commun . 4:1922 doi: 10.1038/ncomms2944 (2013).